Asymmetric synthesis ofP-stereogenic phosphindane oxides via kinetic resolution and their biological activity The importance of P -stereogenic heterocycles has been widely recognized with their extensive use as privileged chiral ligands and bioactive compounds. The catalytic asymmetric synthesis of P -stereogenic phosphindane derivatives, however, remains a challenging task. Herein, we report a catalytic kinetic resolution of phosphindole oxides via rhodium-catalyzed diastereo- and enantioselective conjugate addition to access enantiopure P -stereogenic phosphindane and phosphindole derivatives. This kinetic resolution method features high efficiency (s factor up to >1057), excellent stereoselectivities (all >20:1 dr, up to >99% ee ), and a broad substrate scope. The obtained chiral phosphindane oxides exhibit promising therapeutic efficacy in autosomal dominant polycystic kidney disease (ADPKD), and compound 3az is found to significantly inhibit renal cyst growth both in vitro and in vivo, thus ushering in a promising scaffold for ADPKD drug discovery. This study will not only advance efforts towards the asymmetric synthesis of challenging P -stereogenic heterocycles, but also surely inspire further development of P -stereogenic entities for bioactive small-molecule discovery. P-Stereogenic molecules are widely used as chiral ligands and organocatalysts in organic synthesis [1] , [2] , [3] , [4] , and they are also important structural motifs in pharmaceuticals and biologically active compounds [5] , [6] , [7] . As such, developing efficient methods for asymmetric synthesis of P -stereogenic molecules is an important endeavor in synthetic chemistry [8] , [9] , [10] . Along with the remarkable advances in catalytic asymmetric synthesis of acyclic P -stereogenic molecules [8] , [9] , [10] , [11] , [12] , [13] , [14] , [15] , [16] , [17] , [18] , [19] , [20] , [21] , several catalytic asymmetric strategies such as intramolecular desymmetrization [22] , [23] , [24] , [25] , [26] , [27] and dynamic kinetic cross-coupling [28] , [29] have been successfully developed to generate cyclic P -stereogenic heterocycles. However, the established methods are generally restricted to the construction of 6-memebered or larger P -stereogenic heterocycles [22] , [23] , [24] , [25] , [26] , [27] , [28] , [29] , and the catalytic asymmetric synthesis of 5-membered P -stereogenic heterocycles still remains underdeveloped (Fig. 1a ). In this regard, catalytic asymmetric synthesis of P -stereogenic phosphindanes, which are privileged scaffolds in chiral ligands as exemplified by the powerful BIBOP/DIME-type ligands, DuanPhos, and BeePhos family (Fig. 1b ) [3] , [30] , [31] , [32] , remains a formidable task. Currently, access to enantio-enriched P -stereogenic phosphindanes primarily relies on optical resolution of the racemates using resolving agents or chiral auxiliary-assisted synthesis [33] , [34] . Efforts have been devoted to realizing catalytic asymmetric synthesis of this highly useful chiral scaffold, but construction of the benzo-fused 5-membered-ring can pose huge challenges for controlling the enantioselectivity even though asymmetric synthesis of P -stereogenic phospholanes [35] and dibenzophospholes [36] , [37] has been realized. Glueck achieved a highest 70% ee in the palladium-catalyzed enantioselective intramolecular cyclization of functionalized secondary phosphines or their borane adducts [38] . Recently, Yang developed the copper-catalyzed dynamic kinetic intramolecular cyclization of functionalized secondary phosphine oxides and phosphinates, but the 5-membered product was only obtained with 73% ee while the method showed excellent enantioselectivities in producing 6-membered rings and larger ones [28] , [29] . To the best of our knowledge, the highly enantioselective catalytic synthesis of P -stereogenic phosphindane derivatives has not been developed to date. Fig. 1: P -Stereogenic phosphindane derivatives. a Catalytic asymmetric synthesis of P -stereogenic heterocycles. b Representative P -stereogenic phosphindane derivatives. c Catalytic asymmetric synthesis of P -stereogenic phosphindane derivatives. Full size image Phosphindole oxides are widely used in developing functional materials and their synthesis has been well studied [39] , [40] , [41] . They may serve as readily available precursors for the synthesis of P -stereogenic phosphindane derivatives via a kinetic resolution process, which is a practically useful strategy for accessing challenging chiral scaffold [42] , [43] , [44] , [45] . However, kinetic resolution of phosphindole oxides has not been realized probably due to the difficulties in discriminating the P -stereocenter that is away from the potential reaction site. As part of our continued interest in asymmetric synthesis via remote stereocontrol under rhodium catalysis [46] , [47] , [48] and inspired by Hayashi’s work on rhodium-catalyzed asymmetric synthesis of P -stereogenic phospholanes [35] , we envisaged that the remote P -stereocenter of phosphindole oxides might be effectively discriminated by a suitable chiral rhodium catalyst, which can be employed for kinetic resolution of racemic P -stereogenic phosphindole oxides. Here, we disclose the successful kinetic resolution of phosphindole oxides via rhodium-catalyzed asymmetric conjugate addition for the asymmetric synthesis of P -stereogenic phosphindane oxides and phosphindole oxides. In addition, the P -stereogenic phosphindane oxides are found to exhibit promising therapeutic efficacy in autosomal dominant polycystic kidney disease (ADPKD), which discloses phosphindane derivative a promising scaffold in drug development (Fig. 1c ). 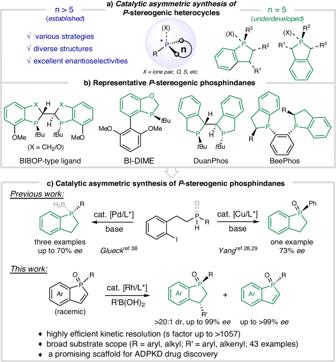Fig. 1:P-Stereogenic phosphindane derivatives. aCatalytic asymmetric synthesis ofP-stereogenic heterocycles.bRepresentativeP-stereogenic phosphindane derivatives.cCatalytic asymmetric synthesis ofP-stereogenic phosphindane derivatives. Reaction development We initiated our investigation by exploring rhodium-catalyzed asymmetric arylation of racemic phosphindole oxide 1a with phenylboronic acid 2a , and the results are summarized in Table 1 . First, the chiral bisphosphine ligands that worked well in the asymmetric arylation of phospholene oxides were tested [35] . To our surprise, the reaction not only produced the conjugate arylation product 3aa , but also gave rise to an unexpected α-arylation product 3aaʹ , and the enantioselectivity was only moderate (entries 1-3). These results clearly indicate that the phosphindole oxide differs from the phospholene oxide in terms of both reactivity and enantio-face recognition. We surmised that the chiral diene ligands, which distinguish from the bisphosphine ligands electronically and sterically [49] , [50] , may match the phosphindole oxide substrate to achieve the desired kinetic resolution. Indeed, the chiral diene ligands exhibited different chemo- and stereoselectivity from bisphosphines in this reaction. As exemplified by entry 4 of Table 1 , the chiral diene Ph-bod led to a highly regioselective generation of the conjugate arylation product 3aa ( 3aa : 3aaʹ > 20:1) with 73% ee , and the phosphindole oxide 1a was recovered with 98% ee . Encouraged by this promising result, we examined a series of chiral dienes for this reaction, and the readily available amide-dienes [51] , [52] proved to be the most effective (entries 5–10). All the examined amide-dienes could maintain the excellent regioselectivity (>20:1), and good selectivity was generally achieved (selectivity factor s > 50 for most cases). Among them, the amide-diene L4 bearing a N - t Bu group afforded the best balance of yield and selectivity. Employing L4 as chiral ligand afforded 3aa in 49% yield with 97% ee and enantiopure 1a (>99% ee) in 47% yield (entry 8, s > 211). Other reaction parameters such as the solvent and reaction temperature were also evaluated. The choice of solvent showed to be quite influential on the reaction outcome. For example, the use of 1,4-dioxane only slightly affected the enantioselectivity of 3aa , but the use of toluene led to a much lower yield and a decreased selectivity (entries 11 and 12). When the reaction temperature was lowered, the enantioselectivity was not improved (entry 13). Thus, the reaction parameters of entry 8 were identified as the optimal conditions for the following studies. Table 1 Optimization of resolution of phosphindole oxide 1a a Full size table Substrate scope exploration With the optimal conditions in hand, we then examined the scope of this catalytic kinetic resolution (Fig. 2 ). The model reaction produced chiral phosphindane oxide 3aa (>20:1 dr, 97% ee ) and enantiopure 1a (>99% ee ), and their structures and absolute configurations were determined by single-crystal X-ray diffraction analysis. Arylboronic acids bearing electron-donating substituents ( 3ab - 3ae ), halogens ( 3af - 3ai ), and electron-withdrawing substituents ( 3aj - 3al ) at different positions were all suitable for this transformation, delivering the phosphindane oxides in 40-50% yield with 90-99% ee , and the phosphindole oxide 1a was recovered in 42-50% yield with up to >99% ee . Note that a variety of functional groups such as alkenes, halogens and keto carbonyls were tolerated. Arylboronic acids featuring a bulky ortho -substituent still showed high reactivity and selectivity in this catalytic kinetic resolution system ( 3am and 3an ), and the enantiopure phosphindole oxide (>99% ee ) could be recovered in 46% isolated yield. Other arylboronic acids, including the multi-substituted ( 3ao - 3ap ), biphenyl ( 3aq ) and polyaromatic ( 3ar ) ones also worked well to achieve excellent selectivities ( s = 152 to >211). Notably, a range of heteroarylboronic acids can participate in the kinetic resolution reaction with a high level of selectivity ( s > 116 in all the examples) to install different heteroarenes, including indole ( 3as and 3at ), quinoline ( 3au ), (di)benzofuran ( 3av and 3aw ) and (di)benzothiophene ( 3ax and 3ay ). In the case of 3-benzothienylboronic acid, both the phosphindane oxide product ( 3ax ) and the recovered phosphindole oxide ( 1a ) were obtained with >99% ee . This selectivity has touched the upper limit of a kinetic resolution process, showcasing the effectiveness of the current protocol. Besides (hetero)arylboronic acids, alkenylboronic acids also underwent the desired kinetic resolution. A variety of styrylboronic acids with different substituents attached to the phenyl ring gave the corresponding products ( 3az to 3az-5 ) with high selectivity ( s > 75). Cyclic alkenylboronic acid was also compatible with the resolution reaction to achieve a high selectivity ( 3az-6, s > 116). Fig. 2: Substrate scope. Kinetic resolution of phosphindole oxides by Rh-catalyzed asymmetric addition. To a dried Schlenk tube with a magnetic stirring bar were added racemic phosphindole oxide 1 (0.20 mmol), organoboronic acid 2 (0.30 mmol), and [RhCl(L4)] 2 (3.2 mg, 0.004 mmol), followed by the addition of THF (1.0 mL) and aqueous solution of KOH (0.01 mmol in 0.1 mL H 2 O) under N 2 . The reaction mixture was stirred at 70 °C for 20 h under N 2 . Ac acetyl, p -Tol p -tolyl. Full size image The scope of the phosphindole oxides was also explored. When phosphindole oxides bearing diverse substituents at different positions, including 5-position ( 3ba - 3da ), 4-position ( 3ea ), and 6-posistion ( 3fa ) were subjected to the catalytic kinetic resolution, similar or even higher levels of reactivity and selectivity can be achieved. The 7-substiutent led to somewhat lower enantioselectivity of the conjugate addition product ( 3ga ) probably because of steric hindrance, but the phosphindole oxide was recovered with >99% ee . In addition, electron-withdrawing substituents such as CF 3 ( 3 ha ) and NO 2 ( 3ia ) were found to be well tolerated. The impact of P -substitution groups was also examined. Consistent with the aryl substitution, alkyl groups including primary alkyl groups (Me, Et) and bulky alkyl groups (Cy, t Bu) were well tolerated with selectivity factors over 70 ( 3jb - 3ma ). It is worth highlighting that the P - t Bu phosphindole oxide ( 1k ), which is particularly useful in developing chiral phosphine ligand (Fig. 1b , up), can be recovered in 43% yield with >99% ee . Synthetic applications To further demonstrate the practicality of this catalytic system, a 2 mmol-scale kinetic resolution of racemic 1a was carried out, and chiral phosphindane oxide 3aa and enantio-enriched phosphindole oxide 1a could be obtained with the similar efficiency and selectivity as the small scale (Fig. 3a ). The chiral phosphine oxides can be readily reduced, thereby providing the valuable chiral phosphines. As shown in Fig. 3b , reduction of 3aa furnished chiral phosphindane 4 in 96% yield without affecting the diastereo- and enantioselectivity. Double bond was tolerated under the conditions, thus reduction of 3az produced phosphine 5 bearing the olefin moiety, which can serve as a good handle for further derivatization or development of phosphine-olefin hybrid ligand. The enantiopure phosphindole oxide provides a good platform for synthesis of chiral phosphindane derivatives. For example, hydrogenation of ( R )- 1a afforded the enantiopure phosphindane oxide 6 . Moreover, addition of other nucleophiles to ( R )- 1a to generate substituted phosphindane oxide was feasible, as exemplified by the highly diastereoselective addition of diphenylphosphine oxide to generate the enantiopure bisphosphine oxide 7 . Fig. 3: Synthetic utility. a Large scale synthesis. b Derivatization of the P -stereogenic products. Full size image Mechanistic investigations Several mechanistic experiments were carried out to gain preliminary insights into the reaction mechanism. First, ( R )- 1a was applied in the standard kinetic resolution conditions, and only trace amount of the conjugate addition product could be detected (Fig. 4a ). This result indicated that the chiral rhodium catalyst can effectively discriminate the two enantiomers of racemic 1a , thus rendering the high yield and enantioselectivity of the recovered phosphindole oxide. Next, a deuterium labeling experiment was conducted, and the deuteration at the α position likely arose from direct protonolysis of the alkylrhodium species that was generated by the carborhodation step (Fig. 4b ). Finally, the control experiment using N -Me- L4 as the chiral ligand led to a lower yield and a significantly diminished enantioselectivity (Fig. 4c ). This result highlights the importance of the secondary amide moiety in enhancing reactivity and enantioselectivity in this arylation reaction, probably via a H-bonding interaction between the amide-NH and substrate. A plausible mechanism of the rhodium-catalyzed kinetic resolution was proposed based on the experimental results and literature report [53] , [54] . Transmetalation between the active hydroxorhodium catalyst and phenylboronic acids generates the phenylrhodium species, which selectively recognizes ( S )- 1a to undergo the subsequent carborhodation step. The transition state is stabilized by hydrogen bonding interactions between the ligand and the substrate ( TS SR ). Finally, hydrolysis of the alkylrhodium species releases the conjugate addition product and regenerates the hydroxorhodium catalyst (Fig. 4d ). DFT calculation on the carborhodation step, which is decisive for the diastereo- and enantioselectivity of the reaction, was conducted to further understand the observed selectivity. The Gibbs energy differences between competing transition states for the generation of diastereomers are 2.40 kcal/mol ( TS SR vs TS RR ) and 4.86 kcal/mol ( TS SR vs TS SS ), which explains the high diastereoselectivity of the reaction. In addition, a Gibbs energy difference of 5.48 kcal/mol accounts for the high enantioselectivity ( TS SR vs TS RS ). Moreover, the favorable transition state ( TS SR ) is found to be stabilized by hydrogen bonding interactions between the N–H of the ligand and the phosphonyl group of the substrate (see Supplementary Section 2.5 for details). Fig. 4: Mechanistic investigations. a Discrimination of ( R )- 1a by the chiral catalyst. b Deuterium-labeling experiment. c Control experiment. d Proposed catalytic cycle. e DFT study. Full size image Biological activity study Autosomal dominant polycystic kidney disease (ADPKD) is the most common inherited kidney disorder, and discovery of novel and effective therapeutic agents for this disease is urgently needed [55] , [56] . Interestingly, 1-indanone was found to retard cyst development in ADPKD [57] . Considering that phosphindane oxide represents a bioisosteric scaffold of 1-indanone, we thus evaluated the therapeutic potential of these chiral phosphindane oxides on ADPKD treatment. Encouragingly, the selected compounds 3aa, 3ay, 3az and 1a inhibited Madin-Darby canine kidney (MDCK) cell colony formation, indicating their inhibition on epithelial cell proliferation, which is the most important driving force for renal cyst development in ADPKD, and 3az displayed better inhibitory efficacy than others (Fig. 5a ). We then detected the effect of 3az on renal cyst development in different ADPKD models. First, we found that 3az concentration-dependently retarded in vitro MDCK cyst growth (Fig. 5b ) and significantly inhibited renal cyst growth in the ex vivo embryonic kidney cyst model (Fig. 5c ), which are two widely used models to fast evaluate the pharmacological effect of compounds in ADPKD. Furthermore, 3az significantly delayed renal cyst growth in vivo in a rapidly progressive ADPKD mouse model ( Pkd1 flox/flox ;Ksp-Cre mice), as indicated by the decreased KW/BW ratio and cyst area in kidneys (Fig. 5d ). These data demonstrated that 3az significantly inhibited renal cyst growth both in vitro and in vivo, and exhibited a potential therapeutic effect in ADPKD. Notably, 3az showed significantly higher inhibitory effect on renal cyst formation and development of ADPKD than its enantiomer ent -3az (see Supplementary Section 2.6 for details). Finally, to initially elucidate the underlying mechanisms of 3az treatment in ADPKD, we conducted a proteomic analysis of kidney samples from mice with ADPKD and 3az -treated mice with ADPKD. The result revealed main enrichment in microtubule-based process and microtubule cytoskeleton organization (see Supplementary Section 2.7 for details), which were reported to be relevant to the inhibition of renal cyst expansion and cell proliferation [57] . The docking result also showed that 3az could stably bind with tubulin (PDB ID: 6EW0, see Supplementary Section 2.8 for details). Fig. 5: Application of 3az in treatment of ADPKD. a Inhibition of the MDCK cell colony formation. n = 3. p = 0.0063, Con vs 3aa; p = 0.0201, Con vs 3ay; p = 0.0002, Con vs 3az; p = 0.0265, Con vs 1a. One-way ANOVA followed by Dunnett’s post-test. b Concentration-dependent inhibition of the in vitro MDCK cyst growth. n = 3. day 6, p < 0.0001, Con vs 3az 10 μM. 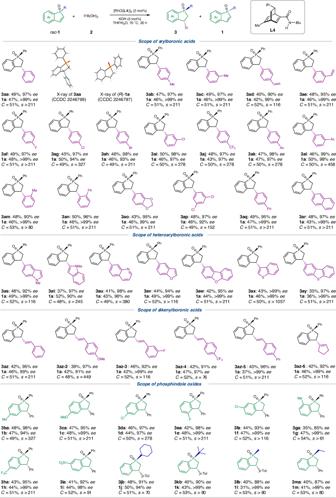Fig. 2: Substrate scope. Kinetic resolution of phosphindole oxides by Rh-catalyzed asymmetric addition. To a dried Schlenk tube with a magnetic stirring bar were added racemic phosphindole oxide1(0.20 mmol), organoboronic acid2(0.30 mmol), and [RhCl(L4)]2(3.2 mg, 0.004 mmol), followed by the addition of THF (1.0 mL) and aqueous solution of KOH (0.01 mmol in 0.1 mL H2O) under N2. The reaction mixture was stirred at 70 °C for 20 h under N2. Ac acetyl,p-Tolp-tolyl. day 8, p = 0.0004, Con vs 3az 1 μM; p < 0.0001, Con vs 3az 10 μM. day 10, p = 0.0013, Con vs 3az 1 μM; p < 0.0001, Con vs 3az 10 μM. two-way ANOVA followed by Dunnett’s post-test. c Inhibition of the renal cyst growth in the ex vivo embryonic kidney cyst model. n = 3. P = 0.0005, Con vs 3az 10 μM. two-sided student’s t test. d Delayed renal cyst grow t h in vivo in a kidney specific Pkd1 knockout mouse model. n = 6. For KW/BW, p < 0.0001. For cyst area, p = 0.0389, Con vs 3az. two-sided student’s t test. Data are presented as mean ± S.E.M., * p < 0.05, ** p < 0.01, *** p < 0.001, **** p < 0.0001. Source data are provided as a Source Data file. Full size image In summary, we have realized the highly enantioselective catalytic synthesis of P -stereogenic phosphindane derivatives by developing a powerful and practical catalytic system that allows the kinetic resolution of racemic phosphindole oxides in high efficiency and enantioselectivity. The flexibility and practicality of the current catalytic system was demonstrated by the broad scope and the large-scale reaction. Moreover, both experimental and computational investigations were conducted to reveal the reaction mechanism, which involves crucial hydrogen bonding interactions between the ligand and the substrate for high stereocontrol. Finally, the chiral phosphindane oxide products were found to exhibit promising therapeutic efficacy in autosomal dominant polycystic kidney disease, which discloses phosphindane a promising scaffold in drug development. This finding shall help expand the chemical space of drug candidates and inspire the discovery of novel leads for drug development. Further investigations on the utility of P -stereogenic phosphindane derivatives in chiral ligand development and drug discovery are currently ongoing in our laboratories. General procedure for the rhodium-catalyzed kinetic resolution of phosphindole oxides To a dried Schlenk tube with a magnetic stirring bar were added racemic phosphindole oxide 1 (0.20 mmol), organoboronic acid 2 (0.30 mmol), and [RhCl(L4)] 2 (3.2 mg, 0.004 mmol), followed by the addition of THF (1.0 mL) and aqueous solution of KOH (0.01 mmol in 0.1 mL H 2 O) under N 2 . The reaction mixture was stirred at 70 °C for 20 h under N 2 . Upon completion, the reaction mixture was diluted with EtOAc (6.0 mL) and water (4.0 mL). The organic layers were separated and the aqueous layer was extracted with EtOAc for two more times (6.0 mL × 2). The combined organic layers were then concentrated in vacuo, and the residue was purified by silica gel chromatography eluting with petroleum ether/THF/EtOH (v/v/v = 80: 20: 1) to give the phosphindane oxide product 3 and the recovered phosphindole oxide 1 . MDCK cell colony formation assay Madin-Darby canine kidney (MDCK) cells were originally obtained from National Collection of Authenticated Cell Cultures (catalog#GNO23). MDCK cells (approximately 800 cells per well) were seeded in 6-well plates and incubated at 37 °C in 5 % (v/v) CO 2 for 24 h. After cell attachment, compounds 3aa, 3ay, 3az, and 1a (10 μМ) were supplemented to the medium and co-cultured for 8 days. Colony formation assays were performed by fixing cells with paraformaldehyde and stained with 0.5 % crystal violet stain solution (Beyotime Biotechnology, Shanghai, China). MDCK cyst model MDCK cells were originally obtained from National Collection of Authenticated Cell Cultures (catalog#GNO23). MDCK cells were seeded in collagen (PureCol, Inamed Biomaterials, Fremont, CA) and mainly induced by 10 μM forskolin (FSK, #F6886, Sigma, Shanghai, China) to form cysts. During a total incubation period of 10 days, compound 3az (0, 1, or 10 μМ) was added to the culture medium from Days 4 to 10. Micrographs of the cysts (at least 10 cysts/well and 3 wells/group) were taken every two days. Cyst diameters were measured and analyzed using ImageView Software (Nexcope, Ningbo, China). Embryonic kidney cyst model All mice were maintained on a C57BL/6 background. C57BL/6 mice were obtained from the animal facility at Xuzhou Medical University. The kidneys of C57BL/6 mice at embryonic Day 13.5 were cultured on Transwells (Corning 3460, NY, USA). Scattered renal cysts formed and progressively expanded in the presence of 100 μM 8-bromoadenosine 3′,5′-cyclic monophosphate (8-Br-cAMP, #B5386, Sigma, Shanghai, China). Compoud 3az (10 μМ) was added to the culture medium to detect the inhibition of cyst formation and growth. Kidneys were photographed using an inverted microscope (Olympus, Tokyo, Japan). The cyst area and total kidney area were measured using Image-Pro Plus 6.0 software (Rockville, MD, USA). ADPKD mouse model All mice were maintained on a C57BL/6 background. Pkd1 flox/flox mice and Ksp-Cre transgenic mice with a C57BL/6 genetic background were obtained from Cyagen (Suzhou, China). To generate Pkd1 flox/− ; Ksp-Cre mice we crossed Pkd1 flox/flox and Ksp-Cre mice. Neonatal mice were genotyped, and the desired genotype (i.e., Pkd1 flox/flox ;Ksp-Cre ) were selected at postnatal day 2. All mice used in this study were 12 days old. 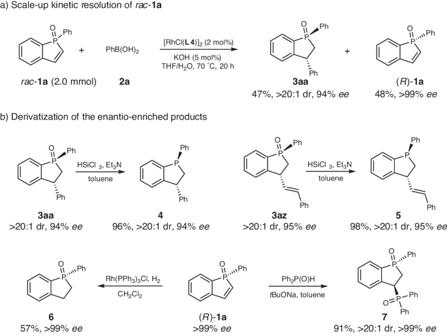Fig. 3: Synthetic utility. aLarge scale synthesis.bDerivatization of theP-stereogenic products. Both male and female mice were used in autosomal dominant polycystic kidney disease (ADPKD) model. Pkd1 was specifically knocked out in the kidney to induce the rapid development of renal cysts in the neonatal period. WT ( Pkd1 +/+ ;Ksp-Cre ) mice and ADPKD ( Pkd1 flox/flox ;Ksp-Cre ) model mice were both divided into 2 groups: a vehicle control group (10% DMSO, 45% saline, 40% PEG300, and 5% Tween80) and 3az -treated group (5 mg/kg d −1 ) ( n = 6). Chemicals were administered to mice by subcutaneous injection on the back every 24 hours from postnatal Day 6 (P6) to P12. The kidneys were harvested and weighed to obtain the kidney index, that is, the ratio of the total kidney weight to body weight (KW/BW). 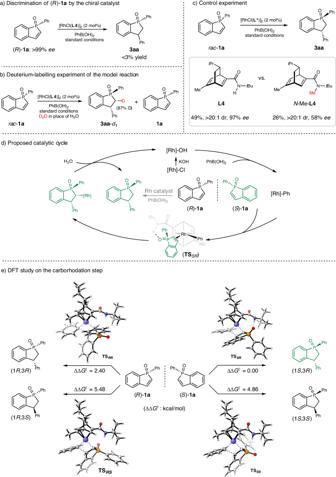Fig. 4: Mechanistic investigations. aDiscrimination of (R)-1aby the chiral catalyst.bDeuterium-labeling experiment.cControl experiment.dProposed catalytic cycle.eDFT study. 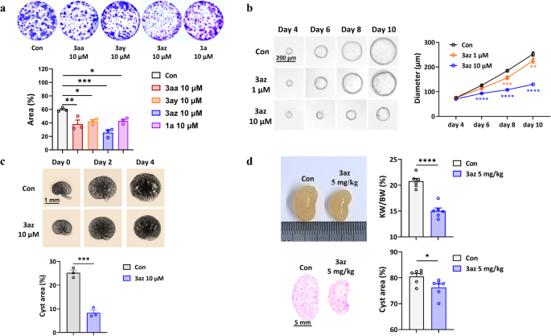Fig. 5: Application of 3az in treatment of ADPKD. aInhibition of the MDCK cell colony formation.n= 3.p= 0.0063, Con vs 3aa;p= 0.0201, Con vs 3ay;p= 0.0002, Con vs 3az;p= 0.0265, Con vs 1a. One-way ANOVA followed by Dunnett’s post-test.bConcentration-dependent inhibition of the in vitro MDCK cyst growth.n= 3. day 6,p< 0.0001, Con vs 3az 10 μM. day 8,p= 0.0004, Con vs 3az 1 μM;p< 0.0001, Con vs 3az 10 μM. day 10,p= 0.0013, Con vs 3az 1 μM;p< 0.0001, Con vs 3az 10 μM. two-way ANOVA followed by Dunnett’s post-test.cInhibition of the renal cyst growth in the ex vivo embryonic kidney cyst model.n= 3.P= 0.0005, Con vs 3az 10 μM. two-sided student’sttest.dDelayed renal cyst growth in vivo in a kidney specificPkd1knockout mouse model.n= 6. For KW/BW,p< 0.0001. For cyst area,p= 0.0389, Con vs 3az. two-sided student’sttest. Data are presented as mean ± S.E.M., *p< 0.05, **p< 0.01, ***p< 0.001, ****p< 0.0001. Source data are provided as a Source Data file. The cyst area and total kidney area were measured using Image-Pro Plus 6.0 software (Rockville, MD, USA). Animal experiments were approved and conducted in accordance with the Laboratory Animal Ethics Committee of Xuzhou Medical University (202309T012). Reporting summary Further information on research design is available in the Nature Portfolio Reporting Summary linked to this article.